Rhodium(II)-catalyzed multicomponent assembly of α,α,α-trisubstituted esters via formal insertion of O–C(sp3)–C(sp2) into C–C bonds The direct cleavage of C(CO)−C single bonds, delivering otherwise inaccessible compounds, is a significant challenge. Although the transition metal-catalyzed insertion of functional groups into C(CO)−C bonds has been studied, strained ketone substrates or chelating assistance were commonly required. In this article, we describe a rhodium(II)-catalyzed three-component reaction of 1,3-diones, diazoesters, and N,N -dimethylformamide (DMF), leading to an unusual formal insertion of O–C(sp 3 )–C(sp 2 ) into unstrained C(CO)−C bonds. This procedure provides a rapid entry to a gamut of otherwise inaccessible α,α,α-trisubstituted esters/amide from relatively simple substrates in a straightforward manner. 55 examples of highly decorated products demonstrate the broad functional group tolerance and substrate scope. The combination of control experiments and isotope-labeling reactions support that O, C(sp 3 ), and C(sp 2 ) units derive from 1,3-diones, diazoesters, and DMF, respectively. Ketones are widely present in natural products and synthetic molecules, and are one of the most fundamental feedstocks in organic synthesis. But while there are many reactions involving the α-functionalization and transformation of carbonyl group of ketones, the selective and catalytic cleavage of C(CO)−C single bonds is still a significant challenge [1] , [2] , [3] , [4] , [5] , [6] , [7] , [8] , [9] , [10] , [11] , [12] , [13] , [14] , [15] , [16] , [17] , [18] , [19] , [20] , [21] , [22] , [23] , [24] , [25] , [26] . Especially, the direct insertion of functional groups into C(CO)−C single bonds, enabling the formation of otherwise inaccessible compounds, is considerably appealing [27] . For example, the traditional Baeyer−Villiger reaction [28] and Büchner−Curtius−Schlotterbeck reaction [29] , [30] , [31] , [32] could directly insert one-atom into C(CO)−C bonds to give esters and homologated ketones, respectively (Fig. 1a ). Recently, transition metal-catalyzed chemoselective insertion of unsaturated units (alkene, allene, alkyne, ketone, and imine) into strained C(CO)−C bonds has been extensively studied by Dong [33] , [34] , [35] , [36] , [37] , [38] , Murakami [39] , [40] , Cramer [41] , [42] , Martin [43] , Chi [44] , and Krische (Fig. 1b ) [45] . However, successful transformation for the catalytic insertion of functional groups into unstrained C(CO)−C bonds is extremely rare, wherein chelating assistance is required [46] . In 2018, Bi and co-workers reported the first example that involve the formal insertion of carbenoids into acyclic C(CO)−C bonds using Ag catalyst (Fig. 1c ) [47] , [48] . Undoubtedly, the development of multiple functional groups, particularly deriving from different molecules, and insertion into unstrained C(CO)−C bonds is of great interest from both practical synthetic applications and mechanistic investigations. Fig. 1: Functional groups insertion into C(CO)−C bonds. a Named reactions involving one-atom insertion into C(CO)−C bonds. b Unsaturated units insertion into strained C(CO)−C bonds. c Ag-catalyzed carbenoid insertion into unstrained C(CO)−C bonds. d Rh-catalyzed insertion of O-C(sp 3 )-C(Sp 2 ) into unstrained C(CO)−C bonds. Full size image In the course of developing transition metal-catalyzed deacylative cross-coupling of 1,3-diones with carbene precursors, we unexpectedly observed the α,α,α-trisubstituted ester products by using N,N -dimethylformamide (DMF) as solvent [49] , [50] , [51] , [52] . Herein we report a multicomponent synthesis of α,α,α-trisubstituted esters from 1,3-diones, diazoesters, and DMF using a rhodium(II) catalyst, in which one-oxygen, one-carbon (sp 3 ), and one carbon (sp 2 ), deriving from 1,3-diones, diazoesters, and DMF, respectively, are inserted into C(CO)−C bonds (Fig. 1d ). This process represents a method for catalytic skeletal remodeling and a complement to cut and sew strategies based on C−C bonds cleavage [27] . 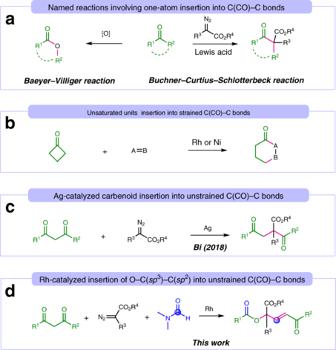Fig. 1: Functional groups insertion into C(CO)−C bonds. aNamed reactions involving one-atom insertion into C(CO)−C bonds.bUnsaturated units insertion into strained C(CO)−C bonds.cAg-catalyzed carbenoid insertion into unstrained C(CO)−C bonds.dRh-catalyzed insertion of O-C(sp3)-C(Sp2) into unstrained C(CO)−C bonds. Reaction development We commenced our study by examining the multicomponent reaction of 1,3-diphenylpropane-1,3-dione ( 1a ), methyl α-phenyldiazoacetate ( 2a ), and DMF in the presence of a catalytic amount of [RuCl 2 ( p -cymene)] 2 at ambient temperature under air atmosphere for 12 h. The three-component reaction product ( 3a ) was obtained in 51% yield (Table 1 , entry 1). The structure of 3a was unambiguously verified by single-crystal X-ray diffraction. We then explored the efficiency of the reaction using different transition metal catalysts. Rh 2 (OAc) 4 and AgOAc catalysts could give the desired product in 65% and 60% yields, respectively (entries 2 and 3), whereas no product was detected using Pd(OAc) 2 and Cu(OAc) 2 catalysts (entries 4 and 5). The choice of Rh salts was also critical to this reaction. 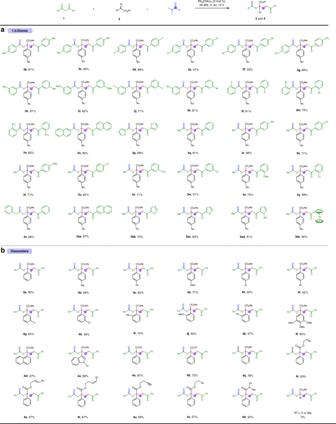Fig. 2: Scope of substrates. aScope of 1,3-diones.bScope of diazoesters. Reaction conditions:1(0.2 mmol),2(0.1 mmol), Rh2(OAc)4(2 mol%), and 4 Å MS (50 mg), in DMF (0.5 mL) at room temperature under air atmosphere for 12 h. Isolated yields based on2are shown. Rh(III) and Rh(I) salts exhibited inferior reactivity compared to Rh(II) salt (entries 6 and 7). A similar yield of 3a was obtained when Rh 2 (esp) 2 was used instead of Rh 2 (OAc) 4 , and no reaction occurred without a catalyst (entries 8 and 9). Remarkably, we noticed that 4 Å MS had a significant effect on the reactivity and gave 3a in 85% yield (entry 10). Further investigation of the loading of catalyst and additive, as well as the concentration of the reaction afforded no better results (entries 11−15). A comparative yield was observed when the reaction was carried out under nitrogen atmosphere (entry 16). Table 1 Optimization of the transition metal-catalyzed C(CO)−C bonds insertion reaction (reaction conditions: 1a (0.2 mmol), 2a (0.1 mmol), catalyst, and additive (50 mg) in DMF (0.5 mL) at room temperature under air atmosphere for 12 h). Full size table Interestingly, the carbenoid insertion (one-carbon insertion) product was not detected in any of the investigations of the reaction parameters [47] , [48] . Substrate scope With the optimized reaction conditions in hand, we explored the substrate scope with respect to 1,3-diones. As shown in Fig. 2a , 1,3-diarylpropane-1,3-diones bearing diverse substituents (methyl, tert -butyl, methoxyl, halogen, and trifluoromethyl) on their aryl rings smoothly underwent reactions to generate the desired α,α,α-trisubstituted esters in 60−97% yields ( 3b − p ). The reactivity of this reaction was slightly influenced by the electronic properties of the aryl rings. 1,3-diarylpropane-1,3-diones with electron-donating groups ( 3b and 3c ) afforded lower yields of the corresponding products than those with electron-withdrawing groups ( 3d − g ). Importantly, the steric hindrance of the aryl rings was not observed to affect the reaction efficiency, and high yields were obtained when substrates with an ortho -substitutent on phenyl rings were used ( 3l − n ). Substrates containing naphthalene and thiophene rings can be successfully converted to the desired products ( 3o and 3p ). Remarkably, aryl alkyl 1,3-diketones delivered the desired products in good to excellent yields with exclusive chemoselectivity, and the C(CO)−C bonds cleavage reactions were found to occur selectively at the alkanoyl−carbon bonds ( 3q − z and 3aa − ae ). It is worth mentioning that the reaction is amenable to a wide range of heteroaryl-substituted 1,3-diones ( 3ab − ad ). Finally, a ferrocene unit could be incorporated into the product with high efficiency ( 3ae ). Fig. 2: Scope of substrates. a Scope of 1,3-diones. b Scope of diazoesters. Reaction conditions: 1 (0.2 mmol), 2 (0.1 mmol), Rh 2 (OAc) 4 (2 mol%), and 4 Å MS (50 mg), in DMF (0.5 mL) at room temperature under air atmosphere for 12 h. Isolated yields based on 2 are shown. Full size image Fig. 3: Gram-scale reaction and functional group transformations. a Gram-scale reaction. b Functional group transformations. Reaction conditions: a 3a (0.1 mmol), LiOH (2 equiv) in THF/H 2 O 4:1 (1 mL) at room temparature. b 3a (0.1 mmol), K 2 CO 3 (2 equiv) in MeOH (1 mL) at room temparature. c 3a (0.1 mmol), NaBH 4 (1.5 equiv) in MeOH (1 mL) at room temperature. d 5a (0.1 mmol), PhNH 2 (1.2 equiv) and TsOH (0.1 equiv) in toluene (1 mL) at 100 °C. Full size image Subsequently, we examined the substrate scope of α-aryldiazoacetates (Fig. 2b ). We first set out to investigate the effect of substituents on the phenyl rings of α-phenyldiazoacetates. A variety of substituted methyl α-phenyldiazoacetates reacted smoothly with 1a , furnishing the desired products ( 4a − l ) in moderated to good yields. The electronic nature of the substituents on the phenyl rings had an obvious effect on the yields, wherein electron-poor groups were less favorable for this reaction ( 4e − h ). In addition, the steric hindrance of the substrates had a negligible effect on the reactivity ( 4i − k ). Moreover, α-naphthyl and α-indolyl diazoacetates were proved to be suitable substrates, giving the corresponding product in 67% and 89% yields, respectively ( 4m and 4n ). We then evaluated the generality of substituents on the ester moieties of α-aryldiazoacetates. Gratifyingly, ethyl, isopropyl, benzyl, allyl, cinnamyl, 3-hexenyl, homopropargyl, and 2-bromoethyl groups were well tolerated, affording the desired products ( 4o − v ) in 57–87% yields. Notably, α-phenyl- N -methyl- N -phenyl diazoacetamide underwent the reaction to provide α,α,α-trisubstituted amide ( 4w ) in 55% yield. Despite the broad substrate scope shown herein (Fig. 2 ), this transformation is not without limitations. For example, when acetylacetone, ethyl acetoacetate, and N -methyl-3-oxobutanamide were subjected to the reaction, no desired products were observed. In addition, the donor−acceptor diazoesters are always required, and α-alkyl and α-H diazoesters failed to give the corresponding products. This might be explained by rapid decomposition of the carbene precursors in the presence of a rhodium(II) catalyst. Synthetic applications This three-component reaction was amenable to a gram-scale synthesis. Ester ( 3a ) could be produced without modifying the standard conditions in 78% yield on a 5 mmol scale (Fig. 3 ). The ester and enone groups of the products of this reaction offer handles for further elaboration. To illustrate this point, several transformations of 3a were studied. First, the 1,4-dione products ( 5a and 5b ) could be obtained via hydrolyzation/decarboxylation/isomerization cascaded reaction from 3a and 3ae , respectively in excellent yields, which could serve as a precursor of Paal–Knorr pyrrole synthesis. Second, treatment of 3a with K 2 CO 3 /MeOH solution led to the transesterification/Micheal addition product ( 6 ) in 90% yield. Moreover, the reduction of 3a with NaBH 4 proceeded efficiently to produce alcohol ( 7 ). Preliminary investigation of reaction mechanism To gain an insight into this Rh-catalyzed C(CO)−C bonds insertion reaction, we performed mechanistic investigations. The reactions were not inhibited by adding 2,2,6,6-tetramethyl-1-piperidinyloxy (TEMPO) or 1,1-diphenylethylene (DPE), which indicated that a radical pathway is unlikely to operate in this reaction system (Fig. 4a ). The result of the reaction of unsymmetrical 1,3-dione ( 1af ) and 2a demonstrated that the chemoselectivity was slightly influenced by the electron density of aryl-groups, and the C(CO)−C bond cleavage tended to occur at the electron-poor moiety (Fig. 4b ). Then, the reaction of 1a and 2a in N , N -diethylformamide was carried out, leading to 3a in 77% yield, whereas no product was formed using N , N -dimethylacetamide as solvent. When N -methyl- N -phenylformamide was used as solvent, 3a and N -methylaniline could be isolated in 21% and 15% yields, respectively (Fig. 4c ). Importantly, the reaction with DMF-formyl- 13 C as solvent gave 3a- 13 C in 86% yield with 99% incorporation (Fig. 4d ). The result of the reaction with DMF-dimethyl- 13 C 2 indicated that the one carbon source could hardly originate from the N -methyl group of DMF (Fig. 4e ). Furthermore, we carried out deuterium-labeling experiments using DMF- D7 (Fig. 4f ). The full incorporation of deuterium was observed at β position of the ester product ( 3a-D-1 ). These results suggest that the formyl group of DMF may serve as the one-carbon source [53] . Next, when the reaction was conducted in the presence of 5 equiv of D 2 O, the incorporation of deuterium at γ position of product ( 3a-D-2 ) was observed (Fig. 4g ). Moreover, 5% of the oxygen atom of ester ( 3q- 18 O-1 ) was labeled using 2 equiv of H 2 18 O, and no 18 O-labeled transesterification/Micheal addition product ( 6 ) was detected (Fig. 4h ). These reactions indicate that water may be generated during the reaction process, and the benzoyl oxygen atom of 3a originates from the in situ generated water. Finally, when the 18 O-labeled 1,3-dione ( 1q- 18 O ) was subjected to the reaction, 22% and 12% of the oxygen atom of 3q- 18 O-2 and 6- 18 O were labeled, respectively, which indicate that the oxygen atom at α position of 3q derives from 1,3-dione (Fig. 4i ). 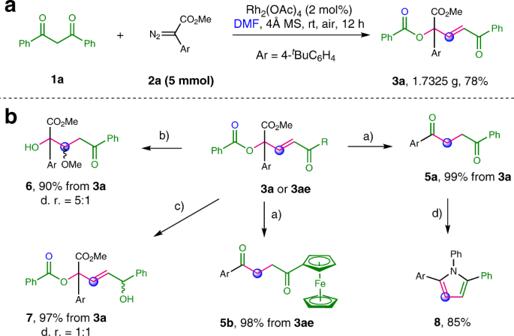Fig. 3: Gram-scale reaction and functional group transformations. aGram-scale reaction.bFunctional group transformations. Reaction conditions:a3a(0.1 mmol), LiOH (2 equiv) in THF/H2O 4:1 (1 mL) at room temparature.b3a(0.1 mmol), K2CO3(2 equiv) in MeOH (1 mL) at room temparature.c3a(0.1 mmol), NaBH4(1.5 equiv) in MeOH (1 mL) at room temperature.d5a(0.1 mmol), PhNH2(1.2 equiv) and TsOH (0.1 equiv) in toluene (1 mL) at 100 °C. Fig. 4: Control experiments and isotope-labeling reactions. a Radical trapping experiments. b The reaction of unsymmetrical 1,3-dione. c The reactions using other amide solvents. d 13 C-labeled experiment using DMF-formyl- 13 C as solvent. e 13 C-labeled experiment using DMF-dimethyl- 13 C 2 as solvent. f Deuterium-labeling experiments using DMF- D7 as solvent. g Deuterium-labeling experiments in the presence of D 2 O. h 18 O-labeled experiment in the presence of H 2 18 O. i The reactions of 18 O-labeled 1,3-dione. Full size image On the basis of the control experiments and literature reports, we proposed a plausible reaction mechanism (Fig. 5 ). Initially, the reaction of α-aryldiazoacetate ( 2 ) with Rh(II) catalyst generates Rh(II) carbene complex ( A ), which is captured by enolate ( B ) to give oxonium ylide ( C ). Then, the nucleophilic addition of oxonium ylide ( C ) to DMF affords aldehyde intermediate ( D ), followed by intramolecular aldol reaction of D , affording the dihydrofuran intermediate ( E ). Finally, intermediate E could be converted into α,α,α-trisubstituted esters ( 3 and 4 ) via a retro -Baylis−Hillman-type reaction. Fig. 5: Plausible reaction mechanism. A plausible mechanism involves the carbene insertion reaction of intermediates A , B to afford oxonium ylide C , subsequent nucleophilic addition, intramolecular aldol reaction, and retro-Baylis−Hillman-type reaction to form the desired products 3 and 4 . Full size image 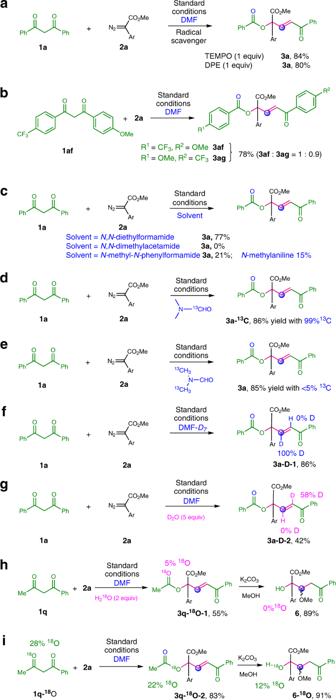Fig. 4: Control experiments and isotope-labeling reactions. aRadical trapping experiments.bThe reaction of unsymmetrical 1,3-dione.cThe reactions using other amide solvents.d13C-labeled experiment using DMF-formyl-13C as solvent.e13C-labeled experiment using DMF-dimethyl-13C2as solvent.fDeuterium-labeling experiments using DMF-D7as solvent.gDeuterium-labeling experiments in the presence of D2O.h18O-labeled experiment in the presence of H218O.iThe reactions of18O-labeled 1,3-dione. 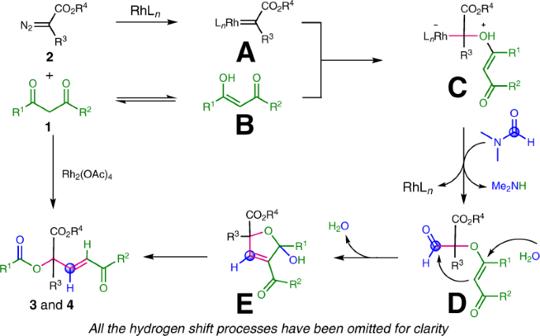Fig. 5: Plausible reaction mechanism. A plausible mechanism involves the carbene insertion reaction of intermediatesA,Bto afford oxonium ylideC, subsequent nucleophilic addition, intramolecular aldol reaction, and retro-Baylis−Hillman-type reaction to form the desired products3and4. In conclusion, we demonstrate an example of Rh(II)-catalyzed formal insertion of O–C(sp 3 )–C(sp 2 ) into unstrained C(CO)–C bonds. A preliminary mechanistic study reveals that O, C(sp 3 ), and C(sp 2 ) units originate from 1,3-diones, diazoesters, and DMF, respectively. This transformation proceeds under mild reaction conditions and opens up a versatile synthetic entry to highly decorated α,α,α-trisubstituted esters/amide from readily accessible starting materials. The development of asymmetric version of this procedure is currently under investigation in our laboratory. General procedure for preparation of 3 A screw-capped reaction vial was charged with 1,3-diones ( 1 ) (0.2 mmol, 2 equiv), methyl 2-(4-( tert -butyl)phenyl)-2-diazoacetate ( 2a ) (23.2 mg, 0.1 mmol, 1 equiv) 4 Å MS (50 mg), and DMF (0.5 mL), followed by the addition of Rh 2 (OAc) 4 (0.8 mg, 0.002 mmol, 2 mol%). The resulting mixture was stirred at room temperature for 12 h, until TLC showed the complete consumption of 2a . After the reaction was completed, the reaction mixture was evaporated under reduced pressure to leave a crude mixture, which was purified by column chromatography on silica gel (eluting with ethyl acetate/petroleum = 1:10) to afford 3 .